Oxidative 1,2-carboamination of alkenes with alkyl nitriles and amines towardγ-amino alkyl nitriles Difunctionalization of alkenes has become a powerful tool for quickly increasing molecular complexity in synthesis. Despite significant progress in the area of alkene difunctionalization involving the incorporation of a nitrogen atom across the C–C double bonds, approaches for the direct 1,2-carboamination of alkenes to produce linear N -containing molecules are scarce and remain a formidable challenge. Here we describe a radical-mediated oxidative intermolecular 1,2-alkylamination of alkenes with alkyl nitriles and amines involving C( sp 3 )–H oxidative functionalization catalysed by a combination of Ag 2 CO 3 with iron Lewis acids. This three-component alkene 1,2-alkylamination method is initiated by the C( sp 3 )–H oxidative radical functionalization, which enables one-step formation of two new chemical bonds, a C–C bond and a C–N bond, to selectively produce γ -amino alkyl nitriles. Difunctionalization of alkenes represents one of the most powerful and straightforward tools to build complex molecules via one-step construction of two chemical bonds that possess significantly synthetic utility in chemical synthesis [1] , [2] , [3] , [4] , [5] , [6] . One of the major synthetic targets for such transformations, including diamination [7] , [8] , [9] , [10] , [11] , [12] , [13] , [14] , [15] , aminooxygenation [16] , [17] , [18] , [19] , [20] , [21] , [22] , [23] , [24] , aminohalogenation [25] , [26] , [27] , [28] , [29] , [30] and carboamination [31] , [32] , [33] , [34] , [35] , [36] , is the incorporation of a nitrogen atom (amino, amide or azide groups) across the C–C double bonds to build useful N -containing molecules through the formation of a C–N bond. Despite significant progress in the field, approaches of the alkene carboamination for producing linear N -containing molecules are scarce and remain a great challenge ( Fig. 1a ): available intermolecular transformations for producing linear N -containing molecules are restricted to the special amination reagents [33] , [34] , [35] , [36] . Further, to our knowledge, three-component carboamination reactions of the alkenes via C–H functionalization have never been reported. 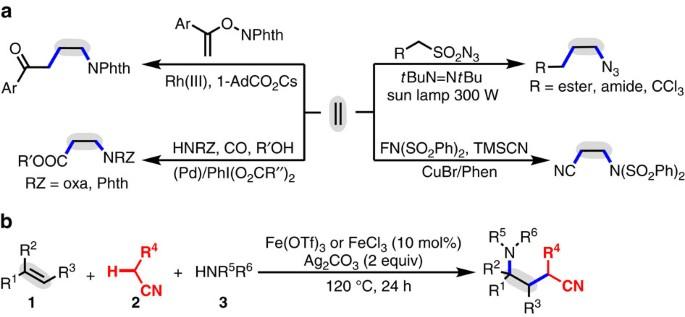Figure 1: 1,2-Carboamination of alkenes. (a) Previous work for 1,2-carboamination of alkenes33,34,35,36. (b) Our radical-mediated three-component, oxidative carboamination between alkenes, alkyl nitriles and amines using a C–H oxidative functionalization. Figure 1: 1,2-Carboamination of alkenes. ( a ) Previous work for 1,2-carboamination of alkenes [33] , [34] , [35] , [36] . ( b ) Our radical-mediated three-component, oxidative carboamination between alkenes, alkyl nitriles and amines using a C–H oxidative functionalization. Full size image In recent years, the C–H oxidative functionalization reaction has attracted much attention due to its inherent features, such as high step economy and atom economy [1] , [2] , [3] , [4] , [5] , [6] , [37] , [38] , [39] , [40] , [41] . Typical transformations include the difunctionalization of alkenes with alkyl C( sp 3 )–H bonds [42] , [43] , [44] , [45] , [46] , [47] , [48] , [49] , [50] , [51] , [52] , [53] , [54] , [55] and the majority of which rely on the formation of a sp 3 -hybridized carbon-centred radical from the oxidative cleavage of the corresponding alkyl C( sp 3 )–H bond followed by addition across the C–C double bond [43] , [44] , [45] , [46] , [47] , [48] , [49] , [50] , [51] , [52] , [53] , [54] , [55] , [56] , [57] , [58] , [59] . However, such approaches are restricted to the 1,2-arylalkylation [52] , [53] , [54] , [55] , [56] , [57] , [58] , [59] , [60] , [61] , [62] , [63] , 1,2-dialkylation [54] and 1,2-oxyalkylation [55] , [56] , [57] , [58] , [59] of the alkenes, and the available three-component transformations are scarce [53] , [55] . In light of these literature results [43] , [44] , [45] , [46] , [47] , [48] , [49] , [50] , [51] , [52] , [53] , [54] , [55] , [56] , [57] , [58] , [59] and our continuous interest in oxidative radical reactions [60] , [61] , [62] , [63] , we envisioned that this C–H oxidative radical functionalization strategy might be viable to achieve 1,2-carboamination of alkenes with new-conceptual, general and straightforward features. Herein, we report an iron-catalysed oxidative three-component 1,2-carboamination of alkenes with alkyl nitriles and amines through C( sp 3 )–H oxidative radical functionalization to assemble γ -amino alkyl nitriles using Ag 2 CO 3 as oxidant ( Fig. 1b ). The reaction enables the simultaneous formation of two new chemical bonds, a C–C bond and a C–N bond, by a sequence of C–H oxidative cleavage, radical addition across the alkenes and aminationin a highly atom-economic and selective manner [64] , [65] , [66] , [67] , [68] . Reaction optimization We initiated the study by investigating various reaction parameters for the three-component reaction of p -methoxystyrene ( 1a ) with acetonitrile ( 2a ) and dibenzylamine ( 3a ) ( Table 1 ). A combination of 10 mol% Fe(OTf) 3 , 2 equiv Ag 2 CO 3 , 120 °C and 24 h were found as the optimal reaction conditions for the conversion of alkene 1a , nitrile 2a and amine 3a to the desired product 4 in 82% yield (entry 1). The results suggest that Ag 2 CO 3 is the real catalysts and Fe(OTf) 3 only serves as a Lewis acid to promote the reaction (entries 2 and 3): although in the absence of Fe(OTf) 3 transformation of alkene 2a to 4 took place albeit giving a lower yield (entry 2), no desired reaction was observed without Ag salts (entry 3). Other Ag salts, including Ag 2 O, AgOAc and AgNO 3 , had the catalytic activity for the reaction, but they were less effective than Ag 2 CO 3 (entries 4–6). Among the amount of Ag 2 CO 3 examined, the use of 2 equiv was turned out to be preferred (entries 1, 7 and 8). Encouraged by these, a series of other Lewis acids, such as FeCl 3 , Yb(OTf) 3 , Cu(OTf) 2 and In(OTf) 3 , were tested (entries 9–12): they could improve the reaction, but were less effective than Fe(OTf) 3 . Notably, the use of other bases, Na 2 CO 3 or Cs 2 CO 3 , instead of Ag 2 CO 3 , resulted in no formation of product 4 (entries 13 and 14), suggesting that Ag 2 CO 3 may act as an oxidant and a catalyst, not a base. Notably, the reported efficient oxidative systems, t BuOO t Bu di- tert -butyl peroxide (DTBP) [42] , [43] , [44] , [45] , [46] , [47] , [48] , [49] , [50] , [51] , [52] , [53] , [54] , [55] or Ag 2 CO 3 /K 2 S 2 O 8 (refs 60 , 61 , 62 , 63 , 64 , 65 , 66 , 67 ) displayed rather lower activity for the reaction (entries 15 and 16). We found that the reaction was sensitive to the temperatures (entries 17 and 18): a lower temperature (100 °C) had a negative effect on the reaction, whereas a higher temperature (130 °C) did not improve the yield compared with the results at 120 °C. Gratifyingly, the reaction could be successfully performed in PhCF 3 medium (entry 19). Table 1 Screening of optimal reaction conditions. Full size table Substrate scope with amines and amides We next explored the scope of this Ag 2 CO 3 -mediated 1,2-carboamination protocol under the optimal reaction conditions with regard to alkenes 1 , nitriles 2 and amines 3 ( Tables 2 and 3 ). 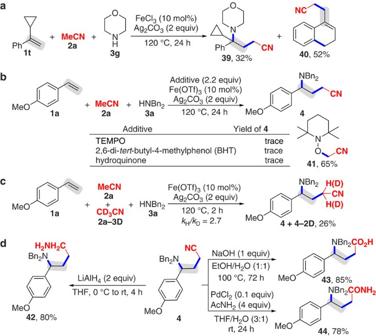Figure 2: Control experiments and utilizations of product 4. (a) Radical testing experiment based on the selectivity. (b) Trapping experiments with a stoichiometric amount of radical inhibitors. (c) Kinetic isotopic effect (KIE) study. (d) Synthetic utilizations. We first turned our attention to investigate the applicability of the optimal conditions in the reaction with various amines 3b–m in the presence of alkene 1a and acetonitrile 2a ( Table 2 ). The resulted indicated that a wide range of secondary and primary amines 3b–j were smoothly converted to the desired products 5–13 in moderate to good yields. N -Methyl-1-phenylmethanamine ( 3b ) was viable to furnish 5 with 89% yield in the presence of Fe(OTf) 3 and Ag 2 CO 3 . For other amines 3c–j , however, Fe(OTf) 3 displayed less efficient than FeCl 3 (products 6–13 ): although treatment of alkene 1a with nitrile 2a , diisopropylamine ( 3c ), Fe(OTf) 3 and Ag 2 CO 3 afforded 6 in 56% yield, the use of FeCl 3 instead of Fe(OTf) 3 enhanced the yield to 66%. Similarly, the yield of 10 from the reaction with morpholine ( 3g ) increased from 74 to 83% when using FeCl 3 instead of Fe(OTf) 3 . To our delight, the optimal conditions were compatible with sulfonamides 3e , 3k and 3l , giving products 8 , 14 and 15 in high yields. Unfortunately, attempt to difunctionalization with acetamide 3m failed to build 1,2-carboamination product 16 . Table 2 Variation of the alkyl nitriles (2) and amines (3). 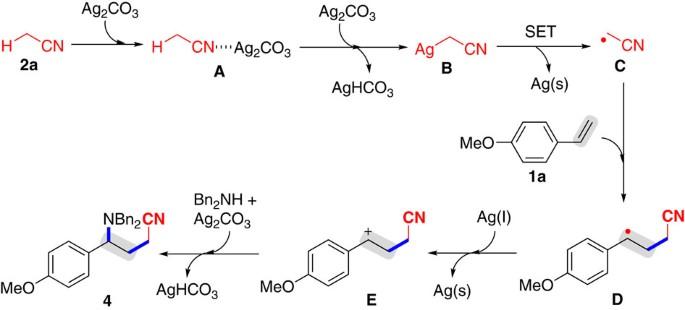Figure 3: Possible mechanism. The alkyl radicalCis generated from decomposition of the AgCH2CN intermediateBvia single-electron transfer. Subsequently, addition of the alkyl radicalCacross the C–C double and oxidative amination afford product4. Full size table Table 3 Variation of the alkenes (1). Full size table Subsequently, the scope of alkyl nitriles 2 was exploited in the presence of alkene 1a , morpholine 3g , FeCl 3 and Ag 2 CO 3 ( Table 2 ). In the case of butyronitrile 2b , the reaction afforded 17 in 66% yield. Gratifyingly, the reaction was well tolerated of various acetonitriles 2c–e bearing a Ph group, a MeO group or a CO 2 Et group at the α position, generating 18 – 20 in 50–70% yields. An interesting observation was that secondary alkyl nitrile 2f containing a cyclohexyl ring also proceeded the reaction and resulted in the formation of 21 in 58% yield. Substrate scope with alkenes The optimal conditions were applicable to an array of alkenes 1b–f , 1h–i and 1k–s (products 22–26 , 28–29 and 31–38 ), but electron-withdrawing aryl alkene 1g and simple aliphatic alkene, namely oct-1-ene ( 1j ), had no reactivity (products 27 and 30 ; Table 3 ). Initially, the substitution effect of the aryl ring at the terminal alkenes were examined: several substituted aryl rings, such as m -MeOC 6 H 4 , o -MeOC 6 H 4 , C 6 H 5 , p -MeC 6 H 4 , m -MeC 6 H 4 , naphthalen-2-yl and 3-methylthiophen-2-yl, were perfectly tolerated, and both the electronic nature of the aryl group and the substituent position on the aryl group had an impact on the reactivity (products 22–29 ). Using m -methoxystyrene ( 1b ), for example, afforded 22 in 55% yield, whereas bulky o -methoxystyrene ( 1c ) furnished 23 in 76% yield. Alkene 1f having a weak electron-deficient 4-ClC 6 H 4 group successfully underwent the 1,2-alkylamination reaction to offer 26 , albeit in a diminished yield. However, alkene 1g having a strong electron-deficient 4-CNC 6 H 4 group had no reactivity (product 27 ). Gratifyingly, the optimal conditions were consistent with 1,1-disubstituted alkenes, including 1,1-diphenylethylene ( 1k ), prop-1-en-2-ylbenzene ( 1l ), 1-methoxy-4-(3-methylbut-3-en-1-yn-1-yl)benzene ( 1m ) and 1-methylene-1,2,3,4-tetrahydronaphthalene ( 1n ), generating 31–34 with concomitant formation of a quaternary carbon centre. A particularly attractive feature of this 1,2-alkylamination is the ability to enable the conversion of di- and trisubstituted internal alkenes 1o–s to diverse complex products 35–38 in moderate to good yields. It was noted that the reaction of ( E )-1-methoxy-4-(prop-1-en-1-yl)benzene ( 1o ) or ( Z )-1-methoxy-4-(prop-1-en-1-yl)benzene ( 1p ) had no retention of geometrical selectivity in the double bond (product 35 ), which supported a radical process. Control experiments and mechanistic studies Using (1-cyclopropylvinyl)benzene ( 1t ) to react with nitrile 2a and amine 3g , the 1,2-alkylarmination product 39 along with the mono alkylation/ring-opening/cyclization product 40 was observed ( Fig. 2a ) [55] . Notably, the reaction of alkene 1a with nitrile 2a and amine 3a could not take place in the presence of a stoichiometric amount of radical inhibitors, such as 2,2,6,6-Tetramethyl-1-piperidinyloxy (TEMPO), 2,6-di- tert -butyl-4-methylphenol and hydroquinone ( Fig. 2b ). Figure 2: Control experiments and utilizations of product 4. ( a ) Radical testing experiment based on the selectivity. ( b ) Trapping experiments with a stoichiometric amount of radical inhibitors. ( c ) Kinetic isotopic effect (KIE) study. ( d ) Synthetic utilizations. Full size image In addition, under the optimal conditions nitrile 2a reacted with TEMPO afforded product 41 . These results suggested that the current reaction is triggered by a free-radical process. The kinetic isotope effect experiment gave a large kinetic isotope effect value ( k H /k D =2.7), implying that the cleavage of the C( sp 3 )–H bond may be rate-limiting ( Fig. 2c and for the detailed information, see Supplementary Fig. 39 ) [37] , [38] , [39] , [40] , [41] , [42] , [43] , [44] , [45] , [46] , [47] , [48] , [49] , [50] , [51] , [52] , [53] , [54] , [55] . Gratifyingly, product 4 were easily converted to 1,4-diamine 42 , γ -amino acid 43 and γ -amino amide 44 in good yields ( Fig. 2d ) [69] , [70] . Consequently, the mechanisms for the Ag 2 CO 3 -mediated 1,2-alkylamination reaction was proposed ( Fig. 3 ) [31] , [32] , [33] , [34] , [35] , [36] , [37] , [38] , [39] , [40] , [41] , [42] , [43] , [44] , [45] , [46] , [47] , [48] , [49] , [50] , [51] , [52] , [53] , [54] , [55] , [56] , [57] , [58] , [59] , [60] , [61] , [62] , [63] , [64] , [65] , [66] , [67] , [68] . Coordination of the nitrogen atom in MeCN 2a with AgCO 3 gives the intermediate A , which sequentially reacts with AgCO 3 to afford the AgCH 2 CN intermediate B and AgHCO 3 . The decomposition the AgCH 2 CN intermediate B readily takes place under heating to form the alkyl radical C (supported by the results of Fig. 2b ), AgHCO 3 and the Ag 0 species [Ag(s)] through single electron transfer [42] , [43] , [44] , [45] , [46] , [47] , [48] , [49] , [50] , [51] , [52] , [53] , [54] , [55] , [56] , [57] , [58] , [59] , [60] , [61] , [62] , [63] , [64] , [65] . Subsequently, addition of the alkyl radical C across the C–C double bond in alkene 1a produces the alkyl radical intermediate D (supported by the reaction of alkene 1t ; Fig. 2a ). Intermediate D is converted into the carbon-centered cation E , followed by reaction with amine 3a affords the product 4 , AgHCO 3 and the Ag 0 species through a sequence of oxidation and nucleophilic addition [64] , [65] , [66] , [67] , [68] . Notably, the radical intermediates C and D can be stabilized by Lewis acids, thus improving the yields. Figure 3: Possible mechanism. The alkyl radical C is generated from decomposition of the AgCH 2 CN intermediate B via single-electron transfer. Subsequently, addition of the alkyl radical C across the C–C double and oxidative amination afford product 4 . Full size image In summary, we have developed a silver-mediated intermolecular 1,2-alkylamination of alkenes with alkyl nitriles and amines involving C( sp 3 )–H oxidative radical functionalization for producing γ -amino alkyl nitriles. The generality of such an intermolecular 1,2-alkylamination reaction is demonstrated by a wide scope with respect to alkenes, alkyl nitriles and amines. The radical mechanism was also discussed according to the control experiments. Importantly, applications of the products, γ -amino alkyl nitriles, to prepare other valuable synthons have been examined. Currently, our laboratory is working to apply this C–H oxidative radical functionalization strategy in synthesis. General procedure for 1,2-carboamination of alkenes To a Schlenk tube were added Fe(OTf) 3 or FeCl 3 (10 mol%), Ag 2 CO 3 (0.6 mmol), alkene 1 (0.3 mmol), amine 2 (0.6 mmol) and MeCN (2 ml). Then the tube was recharged with argon and the mixture was stirred at 120 °C for 24 h. After cooling to room temperature, the mixture was filtered through a small plug of silica gel to remove the precipitate and washed with with EtOAc (3 × 10 ml). The solvent was then removed in vacuo and the residue was further purified by silica gel flash column chromatography (10–40% ethyl acetate/hexane+0.1% Et 3 N) to afford the desired product. Data availability The X-ray crystallographic coordinates for structures reported in this study have been deposited at the Cambridge Crystallographic Data Centre under deposition number 1453224 ( 4 ). These data can be obtained free of charge from The Cambridge Crystallographic Data Centre via www.ccdc.cam.ac.uk/data_request/cif . All other data supporting the findings of this study are available within the article and its Supplementary Information file or from the authors upon reasonable request. For NMR spectra of the compounds in this article, see Supplementary Figs 1–39 . How to cite this article: Liu, Y.-Y. et al . Oxidative 1,2-carboamination of alkenes with alkyl nitriles and amines toward γ -amino alkyl nitriles. Nat. Commun. 8, 14720 doi: 10.1038/ncomms14720 (2017). Publisher’s note : Springer Nature remains neutral with regard to jurisdictional claims in published maps and institutional affiliations.